Accurate population proxies do not exist between 11.7 and 15 ka in North America 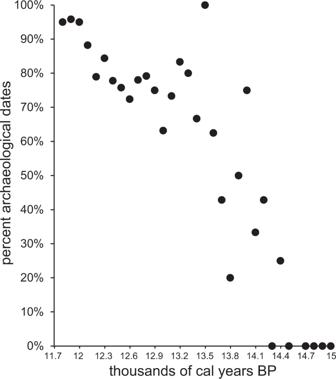Fig. 1: The percentage of archaeological dates associated with human occupation out of all dates in the archaeological dataset used by Stewart and colleagues’2after identifying non-archaeological dates associated with geoarchaeological studies, archaeological sites not widely agreed upon as legitimate, and other questionable contexts. Dates span 11.7 to 15 ka and are binned in 100 year intervals using the median calibrated age estimate. Archaeological radiocarbon dates grow increasingly uncommon toward the past in the dataset used by Stewart and colleagues2, which has falsely extended the age of human occupation and overestimated human abundance for the earliest portions of the analysis. Further information on research design is available in the Nature Research Reporting Summary linked to this article.